Electrically controllable spontaneous magnetism in nanoscale mixed phase multiferroics Magnetoelectrics and multiferroics present exciting opportunities for electric-field control of magnetism. However, there are few room-temperature ferromagnetic-ferroelectrics. Among the various types of multiferroics the bismuth ferrite system has received much attention primarily because both the ferroelectric and the antiferromagnetic orders are quite robust at room temperature. Here we demonstrate the emergence of an enhanced spontaneous magnetization in a strain-driven rhombohedral and super-tetragonal mixed phase of BiFeO 3 . Using X-ray magnetic circular dichroism-based photoemission electron microscopy coupled with macroscopic magnetic measurements, we find that the spontaneous magnetization of the rhombohedral phase is significantly enhanced above the canted antiferromagnetic moment in the bulk phase, as a consequence of a piezomagnetic coupling to the adjacent tetragonal-like phase and the epitaxial constraint. Reversible electric-field control and manipulation of this magnetic moment at room temperature is also shown. The ability to use epitaxy to control the ground state of a material has enabled the discovery of a wide range of new phenomena in modern materials [1] , [2] . Recently, large compressive epitaxial strains were imposed on the rhombohedral phase (R-phase) multiferroic BiFeO 3 (BFO) to stabilize a tetragonal-like phase (T-phase) with a significantly larger c/a ratio [3] . It was also demonstrated that partial relaxation of this epitaxial strain leads to the formation of a nanoscale mixture of the T- and R-phases, thus resembling a classical morphotropic phase boundary in modern piezoelectrics [4] , [5] . Over the past two decades, novel physical phenomena have emerged in complex oxides at interfaces that are naturally created within the system (e.g., phase-separated manganites, relaxor ferroelectrics), or in artificially engineered heterostructures [6] , [7] , [8] , [9] , [10] , [11] . Although many of these phenomena have emerged as a consequence of chemical substitutions, strain control is emerging as an equally powerful tool to create and manipulate such phenomena [2] . In this study, we describe a novel approach to create a new magnetic state in BFO, and we electrically control this emergent magnetism at room temperature. An enhanced spontaneous magnetization arises in the R-phase that is strain confined between T-phases. We demonstrate that this local magnetic moment can be erased by the application of an electric field. Finally, reversal of the electric-field polarity restores the mixed phase structure [12] , [13] . Structure characterization and analysis The samples were prepared using pulsed laser deposition in conjunction with high-pressure reflective high-energy electron diffraction to monitor the growth of the BFO thin films. A bottom conducting layer of LaNiO 3 was inserted to eliminate charging effects during X-ray illumination. 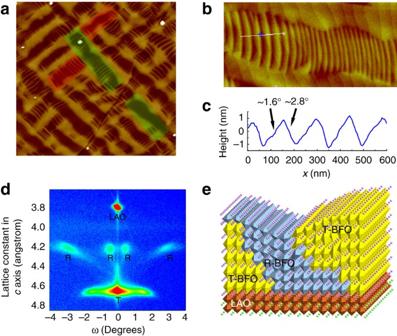Figure 1: Understanding the structures of different phases in mixed phase BFO thin films. (a) Atomic force microscopy topography image of mixed phase BFO sample. Red and green shaded areas indicate two sets of mixed phase features oriented at 90° to each other. (b) High-resolution atomic force microscopy topography image of a mixed phase structure. (c) Cross-section line profile along the white line in (b). R- and T-phases show different slopes of∼1.6° and∼2.8°. (d) X-ray diffraction 2θ-ωmap of a mixed phase film. (e) Schematic of T/R mixed phase structure. LAO, LaAlO3. Partial strain relaxation through control of the film thickness leads to the formation of two orthogonal arrays of nanoscale, T+R phase mixtures, as imaged by atomic force microscope (AFM) shown in Figure 1a . The individual stripe-like regions, Figure 1b , consist of a nanoscale ensemble of T- and R-phases with a characteristic length scale of 20–40 nm. The graph in Figure 1c shows a cross-sectional line-profile of the mixed phase area, revealing two different tilting angles (2.8° and 1.6° relative to the surface plane) of the mixed phase areas. The structural details of such a mixed phase ensemble were identified from careful X-ray diffraction 2 θ - ω scans, such as that shown in Figure 1d . The X-ray data also identifies the structural distortion of the R-phase, with out-of-plane lattice parameter of ( c =4.17 Å); this coupled with reciprocal space maps provides a measure of the in-plane dimensions of this highly strained R-phase to be 3.82 Å. From the four peaks arising from the R-phase, Figure 1d , the tilt angles for these can be divided into two groups, one ∼ 2.8° and the other ∼ 0.6°, which correspond to the green and red shaded areas in Figure 1a . The broadening angle for the T-phase (c=4.64 Å) is estimated to be 1.6°, resulting from the tilting of the T-phase, consistent with the AFM measurement. Compared with the AFM line profile, we find that the T-phase with a tilt angle of 1.6° is on one side of the peaks and the R-phase with a tilt angle of 2.8° is on the other side of the peaks to the T-phase. Therefore, we can locate the R- and T-phases with the slopes of the topography shown in Figure 1c and schematically illustrated in Figure 1e . The AFM and X-ray diffraction studies clearly establish the nanoscale, R–T mixed-phase ensemble, in which the R-phase is highly strained compared with the bulk. As BFO in the bulk is a well-known ferroelectric and canted antiferromagnet [14] , [15] , [16] , it is natural to ask: what is the magnetic state of the mixed phase BFO, especially in the highly strained R-phase? Figure 1: Understanding the structures of different phases in mixed phase BFO thin films. ( a ) Atomic force microscopy topography image of mixed phase BFO sample. Red and green shaded areas indicate two sets of mixed phase features oriented at 90° to each other. ( b ) High-resolution atomic force microscopy topography image of a mixed phase structure. ( c ) Cross-section line profile along the white line in ( b ). R- and T-phases show different slopes of ∼ 1.6° and ∼ 2.8°. ( d ) X-ray diffraction 2 θ - ω map of a mixed phase film. ( e ) Schematic of T/R mixed phase structure. LAO, LaAlO 3 . Full size image Magnetic characterization and analysis X-ray magnetic circular dichroism (XMCD) is a powerful method to study the magnetic response of a material [17] , [18] . We have used this technique to explore the magnetic response of BFO films with mixed phases, and compared with unconstrained R- and pure T-phase films. X-ray absorption spectra at Fe 3+ L 2,3 -edge using left and right circularly polarized (RCP) soft X-rays, at grazing incidence ( θ =30°) were obtained as a function of the external magnetic field in total electron yield mode. 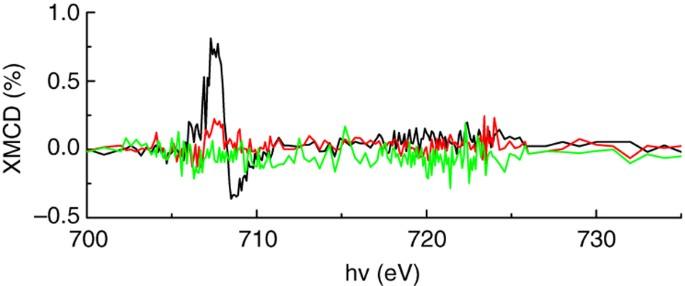Figure 2: X-ray magnetic circular dichroism study of different phases. Mixed phase (black), pure rhombohedral phase (red) and pure tetragonal phase films (green). Fe L3,2XMCD spectra of BFO films in the three different phases probed using fixed X-ray circular polarization (right circularly polarized) and point-by-point reversal of the external magnetic field of magnitude 2 T. Figure 2 shows the XMCD signal obtained from the difference between X-ray absorption spectra in positive and negative (parallel and antiparallel to the k -vector of the incident X-ray) magnetic field (±2 T) and fixed X-ray polarization. The red curve in Figure 2 is from a pure R-phase BFO sample, which gives a negligible XMCD signal (as the canted moment is only ∼ 6–8 emu cc −1 ) [14] . No canting of Fe 3+ spins is allowed in the T-phase BFO because of symmetry, and thus, it does not exhibit any XMCD (data in green in Fig. 2 ) [19] . The significantly larger XMCD spectra of mixed T+R phase BFO ensembles are shown as the black curves in Figure 2 , indicating that a higher magnetic moment is present in mixed phase BFO films. The XMCD spectra in Figure 2 are measured with left circularly polarized (LCP) X-rays; they reverse polarity when using RCP X-rays, confirming that the response is magnetic in origin. These measurements clearly reveal the existence of a spontaneous magnetic moment in the mixed phase samples. From the ∼ 0.7% XMCD signal, and using data from other iron oxide systems (Fe 3 O 4 ) [20] , [21] as a semi-quantitative calibration, we estimate the averaged magnetization to be of the order of 20–30 emu ml −1 in the top 5 nm (penetration depth for electrons in total electron yield mode) of the sample surface. To explore the microscopic origins of this enhanced magnetic moment, the XMCD signal was imaged using photoemission electron microscopy (PEEM). Figure 2: X-ray magnetic circular dichroism study of different phases. Mixed phase (black), pure rhombohedral phase (red) and pure tetragonal phase films (green). Fe L 3,2 XMCD spectra of BFO films in the three different phases probed using fixed X-ray circular polarization (right circularly polarized) and point-by-point reversal of the external magnetic field of magnitude 2 T. Full size image Spatially resolved PEEM images were obtained using both LCP and RCP incident X-rays at a grazing incidence angle ( θ =30°). To enhance the difference in the magnetic contrast and eliminate the contribution from the topographic contrast, the ratio of the two images was taken. The image contrast is effectively a map of the local magnetization vector; regions that have their magnetic moment lying parallel to the X-ray wave vector show bright contrast, whereas those that are antiparallel appear in dark contrast. 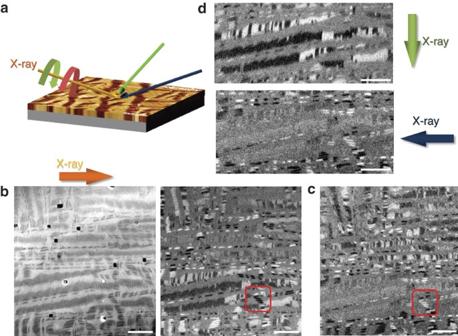Figure 3: Photoemission electron microscopy imaging of a mixed phase film. (a) Schematic of geometry of the measurements. The circularly polarized X-rays indicated by yellow green and blue arrows impinge on the sample at 30° grazing incidence along different crystal orientations. (b) PEEM image in the left panel was obtained from the sum of PEEM image taken with left- and right-circularly polarized X-rays giving topographical contrast. XMCD-PEEM image on the right side showing enhanced magnetic contrast is given from the ratio of PEEM images taken with left and right circularly polarized X-rays at the same location. Black and white contrasts indicate magnetic moments pointing parallel and antiparallel to the incident X-rays. (c) XMCD-PEEM image, showing reversed magnetic contrast, obtained after a sample rotation of 180° as compared withb. (d) XMCD-PEEM images shown on the top and bottom are obtained after a rotation of 90° and 180°, respectively, relative to imageb. Scale bar, 2 μm. XMCD-PEEM images were taken with the incident X-rays at various orientations ( ϕ =0°, 90°, 180°), shown schematically in Figure 3a . Left panel image of Figure 3b is the PEEM image obtained by LCP X-ray at ϕ =0°, showing mainly topographic contrast. The darker areas in this image are the valleys of the mixed phase features and brighter areas are at the peaks. The XMCD image (right panel of Fig. 3b ) reveals the intrinsic magnetic contrast that appears as bright and dark stripe-like patterns indicating that these stripes have magnetic moments lying parallel and antiparallel to the incident X-rays. When the sample is rotated by 180°, all of the stripes reverse contrast, Figure 3c which further confirms the magnetic origin. Moreover, after a 90° rotation of the sample about the sample normal, the stripes show weak or no contrast when the incident X-ray is perpendicular to their long axes; at the same time, the stripes show strongest contrast when the incident X-ray is parallel to their long sides ( Fig. 3d ). These measurements clearly indicate that the magnetic moments in the stripe-like area are lying along the long axis of the stripes. It is also important to note that the regions in bright and dark magnetic contrast in Figure 3b are approximately of equal fractions. Temperature-dependent PEEM studies ( Supplementary Fig. S1 ) show that the magnetic contrast vanishes by ∼ 175 °C, whereas the topography remains unchanged; furthermore, the magnetic contrast re-appears on cooling to room temperature. Figure 3: Photoemission electron microscopy imaging of a mixed phase film. ( a ) Schematic of geometry of the measurements. The circularly polarized X-rays indicated by yellow green and blue arrows impinge on the sample at 30° grazing incidence along different crystal orientations. ( b ) PEEM image in the left panel was obtained from the sum of PEEM image taken with left- and right-circularly polarized X-rays giving topographical contrast. XMCD-PEEM image on the right side showing enhanced magnetic contrast is given from the ratio of PEEM images taken with left and right circularly polarized X-rays at the same location. Black and white contrasts indicate magnetic moments pointing parallel and antiparallel to the incident X-rays. ( c ) XMCD-PEEM image, showing reversed magnetic contrast, obtained after a sample rotation of 180° as compared with b . ( d ) XMCD-PEEM images shown on the top and bottom are obtained after a rotation of 90° and 180°, respectively, relative to image b . Scale bar, 2 μm. Full size image To further explore the origins of the magnetic response (that is, does it arise at the interface between the T/R phases or is it located within the highly strained R-phase), we focus on the area indicated by a red square in Figure 3b,c and compare with both the AFM line scans and the corresponding piezoresponse force microscopy (PFM) images of the same area. 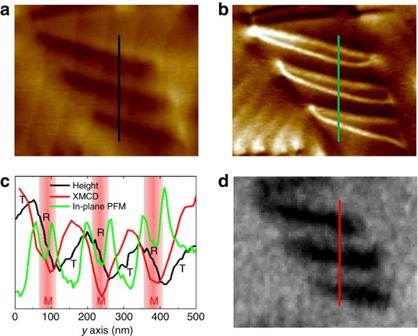Figure 4: Detailed PEEM and PFM analysis of a mixed phase structure. (a,b,d) AFM topography, PFM, high-resolution XMCD-PEEM images of the area indicated by a red box inFigure 3b. (c) Superimposed line profiles of the black, green and red lines indicated ina,bandd. Red shaded areas indicate the enhanced magnetic moment, that is, areas in which the magnitude of XMCD signal reaches its extreme value (minima in XMCD curve). R- and T-phases are labelled next to their corresponding slopes. Figure 4a is the AFM topography image and the corresponding in-plane PFM image acquired simultaneously at exactly the same position is shown in Figure 4b . The PFM image shows bright contrast of 'lip-shaped' patterns surrounding the stripe-like features. By obtaining a line profile across the mixed phase features, the topography curve (black curve in Fig. 4c ) shows a significant asymmetry of slopes on the two sides of the mixed phase stripes similar to what was shown in the cross-sectional AFM line profile in Figure 1b . Combining the in-plane PFM line profile (green curve in Fig. 4c ) with the topology scan helps us to conclude that the lip-shaped patterns form the T/R interface. More importantly, the area enclosed by the 'lip-shaped' region is on the steeper side, which is the R-phase as shown in Figure 1b . The corresponding magnetic information of the same area is obtained from the zoomed-in XMCD-PEEM image, Figure 4d . By superimposing the PEEM and PFM line profiles together in Figure 4c , it is clear that this highly distorted R-phase is the source of the enhanced magnetic moment in the XMCD image, arising from a piezomagnetic effect [22] , [23] , [24] . Figure 4: Detailed PEEM and PFM analysis of a mixed phase structure. ( a , b , d ) AFM topography, PFM, high-resolution XMCD-PEEM images of the area indicated by a red box in Figure 3b . ( c ) Superimposed line profiles of the black, green and red lines indicated in a , b and d . Red shaded areas indicate the enhanced magnetic moment, that is, areas in which the magnitude of XMCD signal reaches its extreme value (minima in XMCD curve). R- and T-phases are labelled next to their corresponding slopes. Full size image Conventional SQUID magnetometry of a large set of mixed phase samples, ( Supplementary Fig. S2 ) yielded an average magnetic moment of ∼ 5 emu cc −1 that is consistently higher than the pure T-phase samples that show moments ∼ 1 emu cc −1 . This moment in the mixed phase can be understood from a careful examination of the AFM and PEEM images coupled with XRD studies. The AFM images show a surface area fraction of the R-phase of ∼ 30–40%; however, careful analysis of 2 θ - ω XRD scans ( Fig. 1d ) yields a volume fraction of the R-phase of ∼ 10–15%, suggesting that the R-phase is tapered towards the substrate. Using this volume fraction information the magnetic moment of the R-phase is estimated to be ∼ 30–50 emu cc −1 , which is consistent with the data we obtained from surface-sensitive XMCD measurements. To further verify the existence of this magnetic moment, we explored the exchange coupling of this moment to a ferromagnetic layer. The 2.5-nm-thick ferromagnetic Co ·90 Fe ·10 (CoFe) thin films were deposited onto BFO films containing a large fraction of mixed phase regions at room temperature by direct-current (DC) magnetron sputtering in a ultra-high vacuum (UHV) system of base pressure of ∼ 5×10 −8 torr. The CoFe films were capped with a 2-nm thick layer of Pt to prevent its oxidation. A uniform magnetic field of 200 Oe was applied during the CoFe growth to set the uniaxial anisotropy direction. Then, Co-edge XMCD-PEEM imaging was used in different orientations (Φ=0°, 45°, 90°, 180°) to investigate the ferromagnetic domain structures of the CoFe layer. 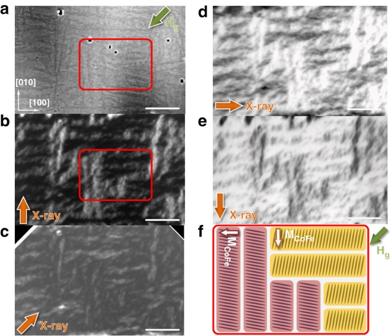Figure 5: Exchange coupling between Co·90Fe·10layer and mixed phase BFO films beneath. (a) LCP-PEEM image of CoFe layer on a mixed phase BFO film showing topographic contrast. The green arrow indicates the direction of applied magnetic field during CoFe growth. (b–e) XMCD-PEEM image obtained from the ratio of LCP and RCP-PEEM images of the same area, showing magnetic contrast of CoFe domains. White, black and grey contrast indicate magnetic moment pointing parallel, antiparallel and perpendicular to the incident X-rays. The direction of incident X-rays is marked by orange arrows. (f) Schematic of magnetic domains in CoFe (wide yellow and purple bars), which simulates the CoFe domain structures of the red-boxed area inaandb, coupled with the mixed phase structure (thin dark ovals) beneath. Magnetic moments of CoFe domains are shown as white arrows. Scale bar, 2 μm. Figure 5a is taken with LCP X-rays, which clearly shows us the topography of mixed phase structure covered by CoFe that was grown in an applied magnetic field along [ ] direction. Bar-shaped magnetic domains can be seen in the XMCD-PEEM images ( Fig. 5b–e ). It is interesting to note that the bar-shaped domain patterns in these magnetic images strongly resemble the corresponding bar-shaped patterns (identified within the red box and schematically depicted in Fig. 5f ) in the topographic image in Figure 5a . Figure 5b was taken with circularly polarized X-rays incident from [010] direction, which shows horizontal bar-shaped domains in dark contrast, whereas vertical bar-shaped domains appear in neutral (grey) contrast, indicating that the magnetization of CoFe in the horizontal and vertical domains are pointing antiparallel ([ ]) and perpendicular ([100] or [ ) to the incident X-rays, respectively. This magnetization direction couples with the moment in the mixed phase features (along the long side of the mixed phase stripes but the short side of the CoFe domains), which is also schematically shown in Figure 5f . When we rotate the sample by 45° with respect to the sample normal, the XMCD amplitude from the CoFe domains decreases by about a factor of √2, reflecting the reduced contrast in the PEEM image shown in Figure 5c . This confirms our interpretation of the moment directions. With a 90° rotation of the sample, the change of contrast of XMCD-PEEM image ( Fig. 5d ) suggests that the moments in the vertical CoFe domains lie along the [100] direction. Finally, a 180° rotation of the sample gives us a fully reversed contrast image ( Fig. 5e ), confirming the contrast we observed here is indeed magnetic in origin and that the moments in the CoFe layer are magnetically coupled to the moment in the R-phase of the BFO underlayer [25] . This robust magnetic coupling provides additional evidence on the existence of magnetic moments embedded in R-phase of the mixed phase nanostructures in BFO. Figure 5: Exchange coupling between Co ·90 Fe ·10 layer and mixed phase BFO films beneath. ( a ) LCP-PEEM image of CoFe layer on a mixed phase BFO film showing topographic contrast. The green arrow indicates the direction of applied magnetic field during CoFe growth. ( b – e ) XMCD-PEEM image obtained from the ratio of LCP and RCP-PEEM images of the same area, showing magnetic contrast of CoFe domains. White, black and grey contrast indicate magnetic moment pointing parallel, antiparallel and perpendicular to the incident X-rays. The direction of incident X-rays is marked by orange arrows. ( f ) Schematic of magnetic domains in CoFe (wide yellow and purple bars), which simulates the CoFe domain structures of the red-boxed area in a and b , coupled with the mixed phase structure (thin dark ovals) beneath. Magnetic moments of CoFe domains are shown as white arrows. Scale bar, 2 μm. Full size image Electrical control of magnetism Having established the existence of a nanoscale magnetic moment in the highly distorted R-phase, we demonstrate the electric-field modulation of this magnetism. By applying a +24 V DC bias to a PFM tip and scanning over the red rectangular area ( Fig. 6a ), the mixed phase features can be transformed into pure T-phase. Then, applying a −8 V DC bias to the green rectangular area, the mixed phase features return. Details of the electric-field-induced phase evolution and the corresponding changes in the piezoresponse are discussed in ref. 26 . 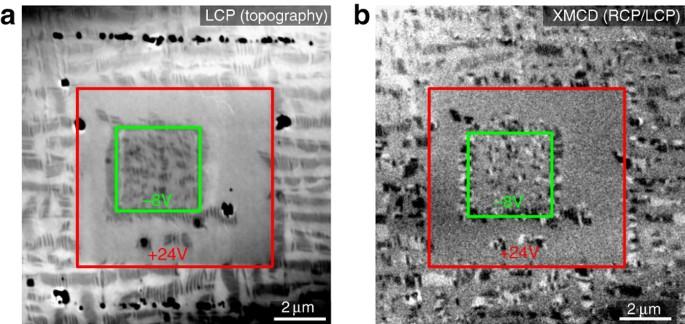Figure 6: Illustration of electrical control of magnetism in mixed phase BFO thin films. (a) LCP-PEEM image of a box-in-box electrically switched area, in which the mixed phase stripes are erased in the area indicated by a red box by scanning with a PFM tip at +24 V DC bias and returned by applying −8 V DC bias in the area indicated by a green area. (b) XMCD-PEEM image of same area as inashowing magnetic contrast from the mixed phase structures. The magnetic moments between the red and green boxes are erased by the electric field and the magnetic moments in the green box are turned on again. LCP and XMCD-PEEM images of this area are shown in Figure 6 . By mapping the magnetic moments (XMCD image), no magnetic contrast is observed in the area between the green and red boxes, consistent with the non-magnetic state of T-phase. In contrast, the XMCD images show the characteristic stripe-shaped features both inside the green box and outside the red box area, indicative of a magnetic moment in them. Therefore, we conclude that magnetic moments in these stripe-shaped nanoscale mixed phase regions can be erased and rewritten at room temperature with only the application of an electric field. Figure 6: Illustration of electrical control of magnetism in mixed phase BFO thin films. ( a ) LCP-PEEM image of a box-in-box electrically switched area, in which the mixed phase stripes are erased in the area indicated by a red box by scanning with a PFM tip at +24 V DC bias and returned by applying −8 V DC bias in the area indicated by a green area. ( b ) XMCD-PEEM image of same area as in a showing magnetic contrast from the mixed phase structures. The magnetic moments between the red and green boxes are erased by the electric field and the magnetic moments in the green box are turned on again. Full size image We have demonstrated a novel approach to manipulate the canted moment of the R-phase of BFO, by creating a nanoscale ensemble in which the R-phase is mechanically confined by regions of the T-phase. This nanoscale mixture displays functional responses that are strikingly different from the parent phases, thus embodying the spirit of a morphotropic phase boundary in a relaxor ferroelectric or the electronically phase-separated scenarios in the CMR manganites. Detailed analyses using a combination of experimental probes reveal that the enhanced magnetic moment resides within the distorted R-phase rather than at the interfaces. The strong coupling to the underlying lattice is a primary reason that this moment is not switchable with a magnetic field; rather, it can be controlled by electric fields that making it a novel vehicle to demonstrate magnetoelectric coupling and electric-field control of magnetism in this multiferroic system. Deterministic control of the location, size and distribution of this mixed phase ensemble would be a critical enabler of approaches to use the results of this study in future magnetoelectronic applications. Pulsed laser deposition Epitaxial thin films of BFO and LaNiO 3 were grown using pulsed laser deposition in conjunction with high-pressure reflective high-energy electron diffraction at 700 °C in 100 mtorr of oxygen. Following deposition of the BFO, the films were cooled in 1 atm of oxygen to room temperature. CoFe deposition The samples were then transported to a vacuum sputtering system with a base pressure of 5×10 −8 torr where the ferromagnetic metal and capping films were grown. Growth of the CoFe films in an applied field, H growth =200 Oe, enables us to induce a uniaxial anisotropy in the system. Then, the CoFe films were capped with a 2-nm thick layer of Pt to prevent its oxidation. Photoemission electron microscopy XMCD-PEEM measurements were completed at various energies and polarizations of focused X-rays that were incident on the sample at an angle of 30° from the surface and formed a spot ∼ 30 μm in diameter. Imaging was done by tuning the photon energy to the Fe L 3 -edge ( ∼ 710 eV) and Co L 3 -edge (~780 eV) and using right- or left-handed circularly polarized radiation enabled imaging of the magnetic moments in both BFO and CoFe by taking the ratio between LCP and RCP images of the same energy at the same location. How to cite this article: He, Q. et al . Electrically controllable spontaneous magnetism in nanoscale mixed phase multiferroics. Nat. Commun. 2:225 doi: 10.1038/ncomms1221 (2011).